Ebf factors and MyoD cooperate to regulate muscle relaxation viaAtp2a1 Myogenic regulatory factors such as MyoD and Myf5 lie at the core of vertebrate muscle differentiation. However, E-boxes, the cognate binding sites for these transcription factors, are not restricted to the promoters/enhancers of muscle cell-specific genes. Thus, the specificity in myogenic transcription is poorly defined. Here we describe the transcription factor Ebf3 as a new determinant of muscle cell-specific transcription. In the absence of Ebf3 the lung does not unfold at birth, resulting in respiratory failure and perinatal death. This is due to a hypercontractile diaphragm with impaired Ca 2+ efflux-related muscle functions. Expression of the Ca 2+ pump Serca1 ( Atp2a1 ) is downregulated in the absence of Ebf3, and its transgenic expression rescues this phenotype. Ebf3 binds directly to the promoter of Atp2a1 and synergises with MyoD in the induction of Atp2a1 . In skeletal muscle, the homologous family member Ebf1 is strongly expressed and together with MyoD induces Atp2a1 . Thus, Ebf3 is a new regulator of terminal muscle differentiation in the diaphragm, and Ebf factors cooperate with MyoD in the induction of muscle-specific genes. Muscle cells in the body of vertebrates specify and differentiate from mesenchymal progenitor cells in the somites [1] . This process is initiated by the combined action of the transcription factors Pax3 and Pax7 (ref. 2 ). Together with the myogenic regulatory factors (MRF) Myf5 and MyoD they form a regulatory network that is central to all early muscle cell differentiation [3] , [4] . Once immature myoblasts have formed, they fuse to generate multinucleated mature muscle cells or myotubes, which constitute the minimal functional unit of all muscles in the body. The transcription factors Myogenin and Mrf4 regulate the later steps of differentiation by influencing the expression of muscle-specific genes encoding contractile proteins in fast and slow twitch fibres [4] . Contraction of skeletal muscles is achieved via the influx of Ca 2+ into the cytosol and its interaction with Troponin C, triggering the ATP-dependent sliding of α-actin and myosin filaments along each other. For relaxation, Ca 2+ is actively removed from the cytosol into the sarcoplasmic reticulum by Serca proteins, which are ATP-dependent Ca 2+ -specific ion pumps [5] , [6] . All MRF proteins bind to E-box sequences that are present in the enhancers or promoters of genes coding for most muscle contractile proteins [4] and also a great many that are not related to muscle-specific genes [7] . Genome-wide Chromatin immunoprecipitation (ChIP)-seq analysis revealed that MyoD binds to a large number of E-boxes including non muscle-specific ones [8] . Therefore, additional transcription factors are required to regulate MRF specificity for particular target genes. Mef2 is such an example, as it binds to sites often present in contractile protein enhancers and interacts cooperatively with MRFs [9] , [10] . Among the skeletal muscles, the diaphragm is one of the most essential ones, separating the pleural and abdominal body cavities. It consists of two different muscles, the crural muscle, which has a central and dorsal location surrounding the oesophagus and aorta, and the costal muscle, which connects the diaphragm’s central tendon to the surrounding ribs. During embryonic development, muscle progenitor cells migrate from cervical somites to the pleuroperitoneal folds, transient structures surrounding the oesophagus [11] . These are assumed to fuse with the septum transversum, which is thought to give rise to the central tendon. Many important aspects of diaphragm development are still unclear, despite its requirement for the unfolding of the lung at birth and subsequent respiration [12] . The family of early B cell factor ( Ebf ) genes encodes a highly homologous group of transcription factors consisting of four members in mammals. The proteins possess a N-terminal DNA-binding domain, which also harbours transactivation potential, followed by an IPT/TIG (immunoglobulin, plexins, transcription factors-like/transcription factor immunoglobulin) domain, presumably mediating protein–protein interaction, and an atypical helix-loop-helix domain required for the formation of homo- and heterodimers. A transactivation domain (TAD) at the C terminus mediates activation of Ebf target genes [13] , [14] . As all four proteins share over 90% sequence homology within these domains, except for the TAD, all Ebf proteins bind to the same DNA sequence and can act redundantly [15] , [16] , [17] . Ebf3 is a member of this protein family that is poorly characterized compared with other Ebf factors. Originally identified in neuronal cells [18] , [19] , Ebf3 is important for cell migration in the developing cortex [17] and in the projection of olfactory neurons to the olfactory bulb [16] . In Xenopus the homologue Xebf3 acts as a regulator of neuronal differentiation downstream of XNeuroD [20] . Furthermore, Ebf3 has been implicated as a negative regulator of cell proliferation [21] . Ectopic expression suppresses proliferation and induces apoptosis of tumour cell lines [22] and Ebf3 was found to be silenced in most high-grade brain tumour cases in a genome-wide screen for tumour suppressors [23] . Silencing of Ebf3 via promoter methylation was also observed in gastric cancer, and ectopic expression induced cell cycle arrest and apoptosis [24] . Here, we present evidence that mammalian muscle cells express Ebf3. Its function is critical in the relaxation of muscle fibres of the diaphragm and essential to allow respiration immediately after birth preventing postnatal lethality. Ebf3 synergises with MyoD in directly regulating the expression of a Ca 2+ pump necessary for muscle relaxation. Thereby, Ebf3 is a new transcription factor involved in the regulation of muscle cell-specific transcription. Expression of Ebf3 To analyse the biological role of Ebf3 , we disrupted its gene locus in murine ES cells. Therefore, a targeting vector was constructed in which an NLS-lacZ gene and a PGK::neo cassette, flanked by loxP sites, were cloned in frame after the translational start codon of Ebf3 , replacing the first four exons of Ebf3 ( Supplementary Fig. 1A ). These exons (representing the first 138 amino acids) encode for essential parts of the DNA-binding and transactivation domain of Ebf3 (ref. 19 ). Two out of 800 clones of mouse embryonic stem cells analysed had correctly incorporated the targeting construction (clones #1 and #2; Supplementary Fig. 1B ). Analysis of genomic DNA from E18.5 embryos from heterozygous matings by PCR revealed the presence of all three possible genotypes ( Supplementary Fig. 1C ; primers indicated in Supplementary Fig. 1A ). To confirm the disruption of Ebf3 independently of the genomic status, semiquantitative RT–PCR was performed, revealing the loss of the Ebf3 transcript in bones of embryonic day (E)18.5 embryos ( Supplementary Fig. 1D ). As a first step in the biological analysis of Ebf3, we determined its expression during embryonic development. Initial but low expression of Ebf3 can be detected in the second branchial arch around E8.5 ( Supplementary Fig. 3A ). Although somites are present at this stage, Ebf3 is expressed in these structures only later, at around E9.0 ( Supplementary Fig. 3B ). In the following stages, the expression of Ebf3 becomes more complex with prominent sites in the midbrain, the branchial arches, the dorsal root ganglia and the olfactory epithelium ( Supplementary Fig. 2 ). To analyse the expression of Ebf3 independently, qPCR was performed on whole wild-type embryos between E7.5 and E18.5 ( Supplementary Fig. 3C ). In this approach, Ebf3 is first detectable at E9.5, strongly increases at E10.5, and is present throughout embryonic development thereafter with a pronounced decrease at E15.5 and E16.5. These results confirm data from EST databases, which list Ebf3 expression from E9.5 on, and are also in line with the β-gal staining shown here, with the only exception that the very first expression was probably below the detection limit in the settings used for qPCR. Furthermore, the data show that the loss of Ebf3 does not alter overall morphology during embryonic development ( Fig. 1a–c and Supplementary Fig. 2 ). A more detailed analysis of tissues and cells in E16.5 embryos reveals prominent expression of Ebf3 in neuronal structures such as the midbrain, the cerebellar primordium and the mantle layer of the spinal cord ( Fig. 1b ). Strong expression is also observed in the olfactory epithelium, adipose tissue and at sites of skeletogenesis such as ribs and vertebrae. Moreover, expression is seen in developing skeletal muscle tissues like the diaphragm and in the limbs. Again, no developmental defects were observed in the absence of Ebf3 ( Fig. 1c ). Staining of E16.5 wild-type embryos indicates the specificity of the observed signals except for the inner lumen of the duodenum ( Fig. 1a ). To quantify the expression of Ebf3 in various tissues, we isolated different organs of E18.5 embryonic and 3-week-old wild-type mice and analysed them by qPCR. Accordingly Ebf3 shows the highest expression in the diaphragm, followed by bone marrow, brain and skeletal muscle in the embryo ( Fig. 1g ). Adult mice express Ebf3 at the highest levels in skeletal muscle followed by the uterus, eye and diaphragm. Intermediate expression levels can be detected in the eye, testis, brain and lymph node, and low expression is seen in the bone marrow and kidney. No expression of Ebf3 was detected in the lung, thymus, spleen, liver and heart ( Fig. 1g ). As diaphragm showed the highest expression among all organs and tissues examined, we analysed its expression in further details using in situ detection of β-galactosidase activity. Ebf3 expression delineates the diaphragm at E18.5, is expressed in the majority, but not all cells ( Fig. 1e ), and is specific in comparison with wild type ( Fig. 1d ). Deletion of one or both alleles of Ebf3 does not change overall morphology, but seems to induce a slightly thickened appearance of the diaphragm ( Fig. 1f ). The diaphragm consists of ~10% type I (slow twitch) and 90% type II (fast twitch) fibres, which can be distinguished by the expression of different isoforms of the myosin heavy chain [25] , [26] . Ebf3 is strongly enriched in cells expressing the type II-associated isoforms MyHC-IIa, MyHC-IIB and MyHC-IIX/D, whereas the type I-associated MyHC-Iβ prevails in Ebf3-negative cells, indicating that Ebf3 is preferentially expressed by type II or fast twitch fibres ( Fig. 1h ). 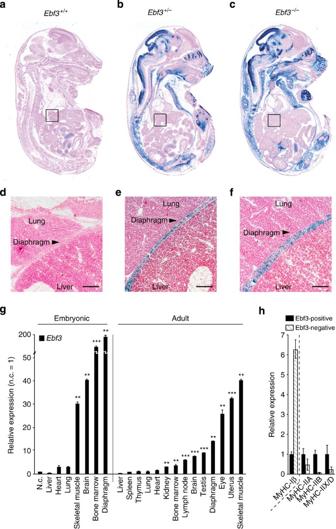Figure 1: Expression ofEbf3at sites of osteogenesis and muscle formation. (a–c) Staining for β-galactosidase in cryosections of E16.5Ebf3+/+(a),Ebf3+/−(b) andEbf3−/−(c) embryos. Ebf3-β-gal-positive cells can be detected in neuronal, olfactory and adipocytic tissues and at sites of osteogenesis and muscle formation. Staining in the lumen of the duodenum is background. (d–f) Magnification of Ebf3-β-gal staining in the area surrounding parts of the diaphragm inEbf3+/+(d),Ebf3+/−(e) andEbf3−/−(f) embryos as indicated by black boxes ina–c. The diaphragm in this magnification is surrounded by the lung and liver tissue as indicated. Bar, 100 μm. (g) Quantitative PCR analysis of the expression ofEbf3in various tissues of wild-type E18.5 embryos (left) or adult animals (right). The pro-B cell line Ba/F3 was used as a negative control and set to 1.n=3; error bars=s.d. Significance is calculated in comparison with BaF/3. **P<0.01, ***P<0.001. (h) Single-cell suspensions from the diaphragm of E18.5Ebf3+/−embryos were sorted into Ebf3-β-gal-positive and -negative cells and subjected to expression analysis of the indicated marker genes for slow (MyHC-Iβ) and fast (MyHC-IIA, MyHC-IIB, MyHC-IIX/D) twitch muscle types by qPCR.n=3; error bars=s.d., *P<0.05 **P<0.01. Figure 1: Expression of Ebf3 at sites of osteogenesis and muscle formation. ( a – c ) Staining for β-galactosidase in cryosections of E16.5 Ebf3 +/+ ( a ), Ebf3 +/− ( b ) and Ebf3 −/− ( c ) embryos. Ebf3-β-gal-positive cells can be detected in neuronal, olfactory and adipocytic tissues and at sites of osteogenesis and muscle formation. Staining in the lumen of the duodenum is background. ( d – f ) Magnification of Ebf3-β-gal staining in the area surrounding parts of the diaphragm in Ebf3 +/+ ( d ), Ebf3 +/− ( e ) and Ebf3 −/− ( f ) embryos as indicated by black boxes in a – c . The diaphragm in this magnification is surrounded by the lung and liver tissue as indicated. Bar, 100 μm. ( g ) Quantitative PCR analysis of the expression of Ebf3 in various tissues of wild-type E18.5 embryos (left) or adult animals (right). The pro-B cell line Ba/F3 was used as a negative control and set to 1. n =3; error bars=s.d. Significance is calculated in comparison with BaF/3. ** P <0.01, *** P <0.001. ( h ) Single-cell suspensions from the diaphragm of E18.5 Ebf3 +/− embryos were sorted into Ebf3-β-gal-positive and -negative cells and subjected to expression analysis of the indicated marker genes for slow (MyHC-Iβ) and fast (MyHC-IIA, MyHC-IIB, MyHC-IIX/D) twitch muscle types by qPCR. n =3; error bars=s.d., * P <0.05 ** P <0.01. Full size image Deletion of Ebf3 leads to respiratory failure Embryonic development proceeds normally in the absence of Ebf3, and, to define the biological role of Ebf3 postnatally, we evaluated genotypes from offspring of heterozygous matings at various time points after birth. From postnatal day 0.5 (D0.5) on, we could not detect any Ebf3 -deficient mice ( Fig. 2a ), and therefore analysed earlier time points observing a normal Mendelian ratio of wild type, heterozygous and knock-out embryos at E18.5 ( Fig. 2a ). This finding suggests lethality around birth, and indeed a close observation of animals at birth revealed that pups were born alive, and Ebf3 −/− mice were indistinguishable from wild-type and heterozygous littermates in their overall appearance. However, immediately after birth, Ebf3 -deficient mice displayed gasping respiration and progressive cyanosis ( Fig. 2b ), and died within 0.5 to 2 h after birth. Examination of wild-type newborn mice showed that the lungs are unfolded and have a normal appearance of alveolar ductal lumens, alveoli and small pulmonary vessels ( Fig. 2c–e , upper row). In contrast, lungs from Ebf3 −/− mice have a congested appearance, do not unfold, and in consequence air-containing passages are not formed as in wild-type lungs ( Fig. 2c–e , lower row). This result suggests that the postnatal lethality and the cyanotic appearance are very likely due to respiratory failure caused by an inability to unfold the lung at birth. However, it seems to be a secondary effect, as Ebf3 is not expressed in the lung ( Fig. 1a–g ), the morphology of the compact lung is normal ( Fig. 2c–e , lower row) and unfolding is not a lung-intrinsic property. 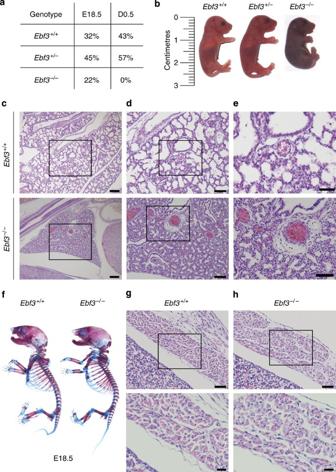Figure 2: Deletion ofEbf3leads to respiratory failure, postnatal death and alterations in muscle morphology. (a) Frequencies ofEbf3wild-type and mutant genotypes before and after birth. NoEbf3-deficient mice can be detected 12 h after birth; E18.5:n=415, D0.5:n=58. (b) Comparison of wild-type (left),Ebf3-heterozygous (middle) andEbf3-deficient (right) newborn mice shortly after birth. Length is indicated in centimetres. (c–e) Histological analysis of longitudinal sections of the lung of wild-type (upper row) andEbf3-deficient (lower row) newborn mice stained with haematoxylin/eosin.dandeare increasing magnifications as indicated by the insets. Bar,c: 200 μm;d: 100 μm;e: 50 μm. (f) Alcian blue/alizarin red staining of cartilage and bone of wild-type orEbf3−/−skeletons at E18.5. (g,h) Cross-sections of diaphragm muscle fibres of newborn wild-type (g) orEbf3-deficient (h) mice stained with haematoxylin/eosin. Lower panels are higher magnifications as indicated by the inset in the upper panels. Bars, upper panels: 50 μm; lower panels: 20 μm. Figure 2: Deletion of Ebf3 leads to respiratory failure, postnatal death and alterations in muscle morphology. ( a ) Frequencies of Ebf3 wild-type and mutant genotypes before and after birth. No Ebf3 -deficient mice can be detected 12 h after birth; E18.5: n =415, D0.5: n =58. ( b ) Comparison of wild-type (left), Ebf3 -heterozygous (middle) and Ebf3 -deficient (right) newborn mice shortly after birth. Length is indicated in centimetres. ( c – e ) Histological analysis of longitudinal sections of the lung of wild-type (upper row) and Ebf3 -deficient (lower row) newborn mice stained with haematoxylin/eosin. d and e are increasing magnifications as indicated by the insets. Bar, c : 200 μm; d : 100 μm; e : 50 μm. ( f ) Alcian blue/alizarin red staining of cartilage and bone of wild-type or Ebf3 −/− skeletons at E18.5. ( g , h ) Cross-sections of diaphragm muscle fibres of newborn wild-type ( g ) or Ebf3 -deficient ( h ) mice stained with haematoxylin/eosin. Lower panels are higher magnifications as indicated by the inset in the upper panels. Bars, upper panels: 50 μm; lower panels: 20 μm. Full size image The diaphragm and the rib cage are necessary to support lung function and breathing, and muscle cells of the diaphragm strongly express Ebf3 ( Fig. 1g ). As osteoblastic cells express Ebf3 during in vitro differentiation [27] , we examined the expression of Ebf3 in bone and bone marrow in vivo to elucidate its role in skeletogenesis and bone formation. The bone marrow is a complex mixture of various cell types, and haematopoietic cells do not express Ebf3 as shown by Ebf3-β-gal staining ( Supplementary Fig. 5A ) or by semiquantitative RT–PCR of E18.5 fetal liver cells ( Supplementary Fig. 5B ). As primary Ebf3-positive mesenchymal cells of the bone marrow express high levels of Scleraxis , aP2 and Prx1 , but no markers of chondrocytes or mature osteoblasts ( Supplementary Fig. 4A ), we conclude that Ebf3 is expressed by immature mesenchymal cells, including mesenchymal stem cells, skeletal progenitors and adipocytes. A slight increase in CFU-F numbers, that is, in the frequency of immature mesenchymal cells of the bone marrow, was observed ( Supplementary Fig. 4B ), but loss of Ebf3 has no effect on the formation of bone and cartilage as exemplified by Alcian blue/Alizarin red staining of E18.5 embryos ( Fig. 2f ) or at various other developmental stages ( Supplementary Fig. 4C ). In addition, analysis of calcified mineral bone by von Kossa staining revealed no differences in the absence of Ebf3 ( Supplementary Fig. 4D ). Furthermore, no defects in fetal haematopoiesis were observed ( Supplementary Fig. 5C ). In contrast, thickening of muscle fibres was observed in the diaphragm of Ebf3 −/− newborn mice, suggesting that deletion of Ebf3 might cause defects in muscle function ( Fig. 2g,h ). Defects in diaphragm contraction in absence of Ebf3 As the diaphragm has a central role in facilitating the unfolding of the lung and supporting breathing after birth [28] , we followed this observation closer. Electron microscopy revealed hypercontracted regions within the diaphragm in the absence of Ebf3 and a shortening of Z-stacks ( Fig. 3A,B ). Within these regions, sarcomere length was reduced 38% from 2.11 μm in wild-type diaphragm to about 1.34 μm in Ebf3 −/− newborn mice ( Fig. 3C ). The phenotype described so far indicates problems with the relaxation of muscle cells in the absence of Ebf3 . To study potential defects in muscle function in more detail, we isolated the diaphragm from Ebf3 wild-type and mutant newborn animals and analysed their reaction to defined electrical stimulation. In a first set of experiments the diaphragm was electrically stimulated with a single pulse of 50 V for 1 ms. Measurement of the resulting twitch shows that the force produced by the Ebf3 -deficient diaphragm was reduced by a factor of 18 compared with wild-type levels ( Fig. 3D ). The total duration of the contraction in response to a single stimulation was prolonged 11.6-fold ( Fig. 3E ). As muscle function normally involves sustained activation, we also measured the same parameters during tetanus stimulation of the isolated diaphragm (50 V, 1 ms, 120 Hz for 500 ms; Supplementary Fig. 6A,B ). The force produced in response to tetanus stimulation was reduced by a factor of 3.6 ( Supplementary Fig. 6A ), confirming data from the single stimulation experiment. Furthermore, the full duration of the contraction after tetanus stimulation was prolonged 23-fold ( Supplementary Fig. 6B ). Taken together, the results indicate a strongly reduced force produced by the diaphragm in response to stimulation, which explains the missing expansion of the lung in Ebf3 -deficient mice and the resulting failure of respiration and cyanotic death. Furthermore, the fact that the muscle can be stimulated, but the duration of the contraction is strongly prolonged, suggests an impairment in muscle relaxation after stimulation. 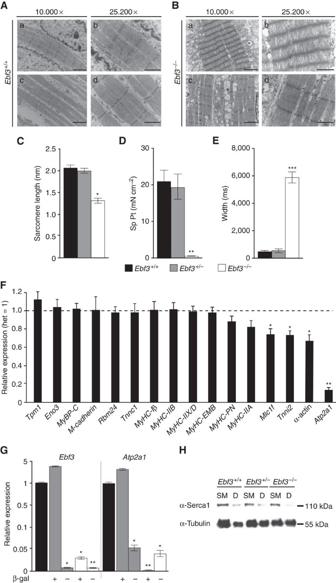Figure 3: Deletion ofEbf3impairs muscle relaxation and expression ofAtp2a1. (A,B) Analysis of the ultrastructure of muscle fibres of the diaphragm by electron microscopy of wild-type (a) andEbf3-deficient (b) newborn mice. Representative electron microscopy pictures of sarcomeres showing myofilaments at 10.000 × (bar, 2.5 nm) and 25.200 × magnification (bar, 1 nm);bshows hypercontracted myofibres. (C) Determination of sarcomere length in the diaphragm ofEbf3+/+,Ebf3+/−andEbf3−/−newborn mice.n=3; error bars=s.d.; *P<0.05. (D,E) Single twitch stimulation (50 V, 1 ms) of diaphragm muscle from newborn mice of the indicated genotypes. (D) Measurement of single twitch normalized to the cross-sectional area, representing muscle force in response to the stimulation. (E) Total duration of muscle contraction after single twitch stimulation.n=5Ebf3+/+,n=7Ebf3+/−,n=4Ebf3−/−; error bars=s.d.; *P<0.05, **P<0.01, ***P<0.001. (F) Ebf3-β-gal-expressing cells were isolated from the diaphragm of E18.5Ebf3+/−embryos by flow cytometry and analysed for the expression of the indicated genes by qPCR. Expression inEbf3+/−cells was set to 1 and relative expression inEbf3−/−cells is shown.n=3, *P<0.05, **P<0.01. (G) Cells of the diaphragm of E18.5 animals were sorted as positive or negative for the expression of Ebf3-β-gal and analysed by quantitative PCR for the expression ofEbf3andAtp2a1. Unsorted cells of wild-type diaphragm were used as control and set to 1;n=3, *P<0.05, **P<0.01. (H) Representative western blot analysis of Serca1 expression in skeletal muscle (SM) and diaphragm (D) of E18.5 embryos of the indicated genotypes;n=3. In all PCR experiments, values are normalized to wild-type levels, error bars represent s.d., andP-values were calculated in comparison to the wild-type control. Figure 3: Deletion of Ebf3 impairs muscle relaxation and expression of Atp2a1 . ( A , B ) Analysis of the ultrastructure of muscle fibres of the diaphragm by electron microscopy of wild-type ( a ) and Ebf3 -deficient ( b ) newborn mice. Representative electron microscopy pictures of sarcomeres showing myofilaments at 10.000 × (bar, 2.5 nm) and 25.200 × magnification (bar, 1 nm); b shows hypercontracted myofibres. ( C ) Determination of sarcomere length in the diaphragm of Ebf3 +/+ , Ebf3 +/− and Ebf3 −/− newborn mice. n =3; error bars=s.d. ; * P <0.05. ( D , E ) Single twitch stimulation (50 V, 1 ms) of diaphragm muscle from newborn mice of the indicated genotypes. ( D ) Measurement of single twitch normalized to the cross-sectional area, representing muscle force in response to the stimulation. ( E ) Total duration of muscle contraction after single twitch stimulation. n =5 Ebf3 +/+ , n =7 Ebf3 +/− , n =4 Ebf3 −/− ; error bars=s.d. ; * P <0.05, ** P <0.01, *** P <0.001. ( F ) Ebf3-β-gal-expressing cells were isolated from the diaphragm of E18.5 Ebf3 +/− embryos by flow cytometry and analysed for the expression of the indicated genes by qPCR. Expression in Ebf3 +/− cells was set to 1 and relative expression in Ebf3 −/− cells is shown. n =3, * P <0.05, ** P <0.01. ( G ) Cells of the diaphragm of E18.5 animals were sorted as positive or negative for the expression of Ebf3-β-gal and analysed by quantitative PCR for the expression of Ebf3 and Atp2a1 . Unsorted cells of wild-type diaphragm were used as control and set to 1; n =3, * P <0.05, ** P <0.01. ( H ) Representative western blot analysis of Serca1 expression in skeletal muscle (SM) and diaphragm (D) of E18.5 embryos of the indicated genotypes; n =3. In all PCR experiments, values are normalized to wild-type levels, error bars represent s.d., and P -values were calculated in comparison to the wild-type control. Full size image Ebf3 is required for expression of Atp2a1 To gain an understanding of the molecular mechanism behind this deficiency, we analysed the expression of genes implicated in muscle contraction and relaxation in the diaphragm of E18.5 wild-type and Ebf3 -deficient mice. The vast majority of these candidate genes did not show differences in expression in absence of Ebf3 ( Fig. 3F ). A slight but significant decrease was observed with Mlc1f , Tnni2 and skeletal muscle-specific α -actin , which are all required for contraction as well as relaxation. Interestingly, the expression of Atp2a1 , which encodes a sarcoplasmic reticulum Ca 2+ -ATPase required for muscle relaxation, was decreased by a factor of ~10, and Ebf3 -deficient mice display an almost exact phenocopy of the deletion of the Atp2a1 gene [29] . As not all cells of the diaphragm express Ebf3 ( Fig. 1e,f ), we sorted Ebf3-β-gal-expressing cells from the diaphragm by flow cytometry from Ebf3 +/− and Ebf3 −/− mice. In heterozygous cells Ebf3 was detected almost exclusively in the β-gal-positive population, showing a high level of purification by this method ( Fig. 3G ). Atp2a1 is a marker for fast twitch muscle cells and was strongly enriched among the Ebf3-β-gal-positive cells in Ebf3 +/− animals, confirming our previous finding that Ebf3 -expressing cells constitute most, if not all, fast twitch type muscle cells of the diaphragm ( Fig. 1h ). In Ebf3 -deficient cells this expression, and thereby the vast majority of overall Atp2a1 expression, was reduced to undetectable levels, whereas a minor level among Ebf3-β-gal-negative cells remained unchanged, indicating a cell-autonomous defect. As expected, Ebf3 expression was reduced to background levels in Ebf3 -deficient cells ( Fig. 3G ). To evaluate whether compensatory mechanisms are active, or whether other members of the Atp2a gene family are also affected by the deletion of Ebf3 , we analysed the diaphragms of E18.5 mice as described [29] . Loss of Ebf3 reduced not only Atp2a1a and Atp2a1b , the two isoforms of Atp2a1 , but also Atp2a2 by a factor of 7.5 and its two isoforms Atp2a2a and Atp2a2b by a factor of 73 and 14, respectively ( Supplementary Fig. 6E ). Conversely, Atp2a3 , the third gene of this family, showed a slight but significant upregulation in absence of Ebf3 ( Supplementary Fig. 6E ). Taken together, loss of Ebf3 leads to a decrease in the expression of the Atp2a1 and Atp2a2 genes and their isoforms, whereas Atp2a3 shows a minor upregulation. The product of the Atp2a1 gene is the Serca1 protein, which has a size of 110 kDa. In Ebf3 -deficient diaphragm, the protein was barely detectable and thus strongly reduced in comparison with wild-type levels ( Fig. 3H ). Quantification of the protein levels indicated a reduction of Serca1 in Ebf3 -deficient diaphragm by a factor of 3.2. In contrast, Serca1 from skeletal muscle did not show a significant reduction in Ebf3 −/− diaphragm compared with Ebf3 +/+ . Atp2a1 rescues Ebf3-dependent respiratory failure Since Ebf3 −/− mice phenocopy Atp2a1 -deficient mice and the expression of Atp2a1 is strongly downregulated in the absence of Ebf3 , we wanted to determine the importance of Atp2a1 as a downstream target of Ebf3. Transgenic animals expressing Atp2a1 under the control of the skeletal muscle-specific skeletal α-actin promoter have been reported [30] . These mice show transgenic expression in skeletal muscles including the diaphragm, but do not have any overt phenotype on their own, allowing us to genetically assess the biological relevance of Atp2a1 as an Ebf3 target gene in vivo . Genotyping of litters from Ebf3 +/− /Atp2a1 tg double-heterozygous crossings revealed a 50% distribution of the Atp2a1 transgene as expected ( Fig. 4a ) from the breeding scheme ( Supplementary Fig. 7 ). Among the Atp2a1 wild-type animals, the frequency of Ebf3 +/+ , Ebf3 +/− and Ebf3 −/− corresponds to the frequency observed previously before and after birth ( Fig. 4a , left panel). In the presence of the Atp2a1 transgene, the ratio of Ebf3 −/− mice at E18.5 surprisingly is not 12.5% as would be expected as a normal Mendelian ratio but 3%, indicating either a genetic interference between Ebf3 and the Atp2a1 transgene or a synthetic phenotype ( Fig. 4a , right panel). We killed mice at stages E12.5 to E16.5, but did not observe a higher percentage of the compound Ebf3 −/− /Atp2a1 tg genotype, arguing against a synthetic phenotype. A defect earlier than E12.5 seems highly unlikely as the skeletal α-actin promoter is not active at these stages. The genomic insertion locus of the Atp2a1 transgene is unknown, but we think the most likely explanation for the low frequency is genetic linkage, that is, the transgene is on the same chromosome as Ebf3 . Strikingly, we observe the same frequency of Ebf3 −/− /Atp2a1 tg animals at D0.5, clearly distinguishing them from Ebf3 −/− mice. Ebf3 −/− /Atp2a1 tg mice do not show any signs of cyanosis or gasping respiration, but display normal morphology and movement at D0.5 ( Fig. 4b ). To determine the level of functional rescue exactly, we analysed sarcomere length in muscle fibres of the diaphragm from Ebf3 +/+ /Atp2a1 tg and Ebf3 −/− /Atp2a1 tg mice and found no significant difference ( Fig. 4c ). Furthermore, we subjected whole diaphragms to defined electrical stimulation as described for the single deletion of Ebf3 . Single twitch stimulation (50 V, 1 ms) induced a force from Ebf3-deficient diaphragms that was comparable to Ebf3-expressing muscle ( Fig. 4d ). In addition, the duration of contraction was also comparable in the diaphragm from Ebf3 +/+ /Atp2a1 tg and Ebf3 +/+ /Atp2a1 tg mice ( Fig. 4e ). The force produced under tetanus stimulation (50 V, 1 ms, 120 Hz for 500 ms) was also rescued by the transgenic expression of Atp2a1 ( Supplementary Fig. 6C ) just as the duration of contraction ( Supplementary Fig. 6D ). Therefore, we conclude that Atp2a1 is the critical target gene downstream of Ebf3 causing the defects in muscle relaxation and the associated cyanotic appearance and postnatal lethality. However, the transgenic expression of Atp2a1 did not allow for prolonged survival of Ebf3 -deficient mice. In a time period from 24 h after birth up to 4 days, all double-mutant mice died, but again did not display a cyanotic appearance ( Fig. 4f ). As Ebf3 −/− /Atp2a1 tg mice seemed slightly weaker and less active over time than their littermates, we determined their weight and found that the gain in newborn mice, particularly from postnatal day 3 on, is not achieved by Ebf3 −/− /Atp2a1 tg mice ( Fig. 4g ). Taken together, the data show that skeletal muscle-specific expression of Atp2a1 rescues the defect in muscle relaxation of the diaphragm, but is unable to compensate for all defects associated with loss of Ebf3 . 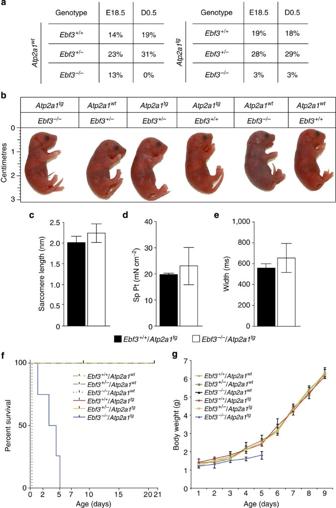Figure 4: Transgenic expression ofAtp2a1rescuesEbf3-dependent respiratory failure. (a)Ebf3-mutant animals were crossed toAtp2a1-transgenic mice and frequencies ofEbf3wild-type and mutant genotypes on an Atp2a1 wild-type or transgenic background are shown before and after birth; E18.5:n=115, D0.5:n=231. (b) Comparison of compoundEbf3-mutant andAtp2a1-transgenic animals as indicated shortly after birth. Note the cyanotic appearance only inEbf3−/−/Atp2a1wtmice;Ebf3−/−/Atp2a1tgmice can be detected 12 h after birth. Length is indicated in centimetres. (c) Determination of sarcomere length in the diaphragm ofEbf3+/+/Atp2a1tgandEbf3−/−/Atp2a1tgnewborn mice.n=3; error bars=s.d. (d,e) Single twitch stimulation (50 V, 1 ms) of diaphragm muscle from newborn mice of the indicated genotypes. (d) Measurement of single twitch normalized to the cross-sectional area, representing muscle force in response to the stimulation. (e) Total duration of muscle contraction after single twitch stimulation.n=3; error bars=s.d. (f) Transgenic expression ofAtp2a1inEbf3-mutant animals does not allow prolonged survival. Survival of animals of the indicated genotypes is followed over time and plotted against days;n= 3 to 5 each. (g) Impaired weight gain in Ebf3-deficient, Serca1 transgenic mice. Animals of the indicated genotypes were weighed every 24 h, and weight is plotted against age of the mice;n=4 to 5 each; error bars=s.d. Figure 4: Transgenic expression of Atp2a1 rescues Ebf3 -dependent respiratory failure. ( a ) Ebf3 -mutant animals were crossed to Atp2a1 -transgenic mice and frequencies of Ebf3 wild-type and mutant genotypes on an Atp2a1 wild-type or transgenic background are shown before and after birth; E18.5: n =115, D0.5: n =231. ( b ) Comparison of compound Ebf3- mutant and Atp2a1 -transgenic animals as indicated shortly after birth. Note the cyanotic appearance only in Ebf3 −/− /Atp2a1 wt mice; Ebf3 −/− /Atp2a1 tg mice can be detected 12 h after birth. Length is indicated in centimetres. ( c ) Determination of sarcomere length in the diaphragm of Ebf3 +/+ /Atp2a1 tg and Ebf3 −/− /Atp2a1 tg newborn mice. n =3; error bars=s.d. ( d , e ) Single twitch stimulation (50 V, 1 ms) of diaphragm muscle from newborn mice of the indicated genotypes. ( d ) Measurement of single twitch normalized to the cross-sectional area, representing muscle force in response to the stimulation. ( e ) Total duration of muscle contraction after single twitch stimulation. n =3; error bars=s.d. ( f ) Transgenic expression of Atp2a1 in Ebf3 -mutant animals does not allow prolonged survival. Survival of animals of the indicated genotypes is followed over time and plotted against days; n = 3 to 5 each. ( g ) Impaired weight gain in Ebf3-deficient, Serca1 transgenic mice. Animals of the indicated genotypes were weighed every 24 h, and weight is plotted against age of the mice; n =4 to 5 each; error bars=s.d. Full size image Atp2a1 is a direct target gene of Ebf3 The biological importance of Atp2a1 downstream of Ebf3 and its downregulation in absence of this transcription factor prompted us to investigate a potential direct molecular link. Atp2a1 maps to mouse chromosome 7 (ref. 31 ), and analysis of DNA sequence upstream of the transcriptional initiation site [32] reveals four potential binding sites for Ebf proteins in its promoter/enhancer ( Fig. 5a ). Two of these possess exactly the same DNA sequence as the Ebf-binding site in the mb-1 promoter where Ebf1 was first identified [33] ; therefore, we named them as M1 and M2, and two sites as E1 and E2, which have the inner palindrome of the ideal consensus site for Ebf proteins [34] . Ebf3 bound with high affinity to the M1 and E2 sites but only weakly to the E1 site as shown by electrophoretic mobility shift assay (EMSA; Fig. 5b ). Ebf3 also bound to the M2 site, but slightly different conditions used for the binding buffer prevent a direct comparison. The binding is specific, as single-nucleotide mutation abolished it (the mutant versions are indicated in Fig. 5a ), and the addition of unlabelled (cold) oligonucleotides in 10-fold excess also leads to a loss of binding activity. Furthermore, the binding activity could be super-shifted by an α-flag antibody, demonstrating complex formation between Ebf3 and the indicated oligonucleotides ( Fig. 5b ). ChIP assay using protein extracts from C2C12 cells expressing flag-tagged Ebf3 showed binding to sites M1, E2 and M2, but not to E1, largely corresponding to the data from the EMSA assay ( Fig. 5c ) and confirming the binding of Ebf3 to these promoter sites in vivo . To determine whether Ebf3 can transactivate from the Atp2a1 promoter via the identified Ebf3-binding sites, a DNA fragment containing over 1 kb of its promoter was cloned into a luciferase reporter construct, and point mutations as indicated in Fig. 5a were introduced into the Ebf-binding sites either alone or in combination. 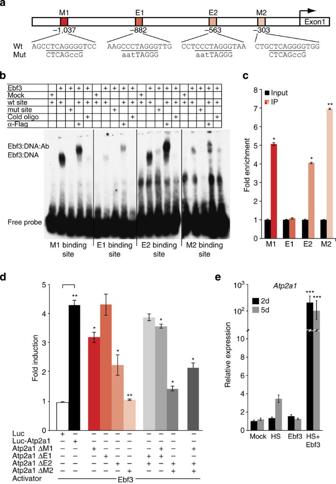Figure 5:Atp2a1is a direct target gene of Ebf3. (a) Schematic overview of the promoter structure of theAtp2a1gene. Red boxes indicate potential binding sites for Ebf proteins, numbers give the position relative to the transcriptional start site ofAtp2a1. The sequence of each potential binding site is indicated and mutations used in the experiments in this figure are shown in small letters. (b) EMSA of HEK293T protein extract containing flag-tagged Ebf3 with oligonucleotides corresponding to potential binding sites. For specificity control non-radioactive (cold) or mutated oligonucleotides were used, identity was confirmed by supershift using α-Flag antibody (Ab);n=3. (c) Chromatin immunoprecipitation (ChIP) of flag-tagged Ebf3 protein from C2C12 cells; qPCR analysis of ChIP using primers specific for all four individual binding sites. Fold enrichment indicates the ratio of DNA amplification comparing ChIP with beads-only control;n=3; error bars=s.d.; *P<0.05, **P<0.01. (d) Analysis of the transactivation potential of Ebf3 from theAtp2a1locus. HEK293T cells were transfected with plasmids comprising all four potential binding sites in wild-type or mutated form as indicated ina. Activity of luciferase was determined, and values were normalized to β-galactosidase. Transfections of the pBL-Luc plasmid not containing promoter elements together with pCMV-Ebf3were set to 1;n=3; error bars=s.d.;P-values were calculated in comparison with activation of pBL-Luc-Atp2a1if not otherwise indicated. *P<0.05, **P<0.01. (e) Quantitative PCR analysis ofAtp2a1expression in C2C12 cells 2 and 5 days after transfection of mock- orEbf3-plasmid and initiation ofin vitrodifferentiation by horse serum (HS).n=3; error bars=s.d.;P-values are relative to mock; ***P<0.001. Figure 5d shows that Ebf3 can transactivate from the Atp2a1 promoter fragment 4.2-fold. Mutation of site M2 almost completely abolished transactivation, whereas mutation of site E1 did not have any influence. Mutation of site M1 or E2 gave intermediary results. Therefore, we conclude that site M2, which is closest to the transcriptional start site, is most important for transactivation of Atp2a1 by Ebf3, and that sites M1 and E2 contribute to reach full activity. Site E1 seems dispensable as Ebf3 binds with low affinity in EMSA, no binding is detected in ChIP assay and transactivation is not influenced by its mutation. In fact, site E1 or neighbouring sequences might negatively influence transactivation, as its deletion together with M1 or E2 results in diminished loss of transactivation ( Fig. 5d ). Finally, to determine whether Ebf3 is not only required but also sufficient for the expression of Atp2a1 , C2C12 cells were transfected with Ebf3 and cultivated in the presence or absence of horse serum to induce myoblast differentiation. Within 2 days, horse serum alone did not induce the expression of Atp2a1 ( Fig. 5e ). Ebf3 alone also had no effect, but in combination with horse serum leads to a strong upregulation of Atp2a1 . After 5 days, Ebf3 had again no effect on the expression of Atp2a1 , and horse serum had a small inductive effect, but together, horse serum and Ebf3 strongly induced the expression of Atp2a1 . These data suggest that Ebf3 alone is not sufficient to induce the expression of endogenous Atp2a1 , but likely acts in concert with other factors expressed during myoblast differentiation. Figure 5: Atp2a1 is a direct target gene of Ebf3. ( a ) Schematic overview of the promoter structure of the Atp2a1 gene. Red boxes indicate potential binding sites for Ebf proteins, numbers give the position relative to the transcriptional start site of Atp2a1 . The sequence of each potential binding site is indicated and mutations used in the experiments in this figure are shown in small letters. ( b ) EMSA of HEK293T protein extract containing flag-tagged Ebf3 with oligonucleotides corresponding to potential binding sites. For specificity control non-radioactive (cold) or mutated oligonucleotides were used, identity was confirmed by supershift using α-Flag antibody (Ab); n =3. ( c ) Chromatin immunoprecipitation (ChIP) of flag-tagged Ebf3 protein from C2C12 cells; qPCR analysis of ChIP using primers specific for all four individual binding sites. Fold enrichment indicates the ratio of DNA amplification comparing ChIP with beads-only control; n =3; error bars=s.d. ; * P <0.05, ** P <0.01. ( d ) Analysis of the transactivation potential of Ebf3 from the Atp2a1 locus. HEK293T cells were transfected with plasmids comprising all four potential binding sites in wild-type or mutated form as indicated in a . Activity of luciferase was determined, and values were normalized to β-galactosidase. Transfections of the pBL-Luc plasmid not containing promoter elements together with pCMV- Ebf3 were set to 1; n =3; error bars=s.d. ; P -values were calculated in comparison with activation of pBL-Luc- Atp2a1 if not otherwise indicated. * P <0.05, ** P <0.01. ( e ) Quantitative PCR analysis of Atp2a1 expression in C2C12 cells 2 and 5 days after transfection of mock- or Ebf3 -plasmid and initiation of in vitro differentiation by horse serum (HS). n =3; error bars=s.d. ; P -values are relative to mock; *** P <0.001. Full size image Ebf3 and MyoD synergistically induce expression of Atp2a1 Other members of the Ebf protein family cooperate with basic helix-loop-helix transcription factors in the induction of target genes, like Ebf1 with E2A in B-cell development [35] , [36] . Moreover, E-boxes, the consensus binding sites for bHLH transcription factors, are found highly enriched in the vicinity of Ebf-binding sites [37] , [38] . A detailed examination of the Atp2a1 promoter yielded five E-boxes within the Atp2a1 promoter fragment (X1–X5, Fig. 6a ). MyoD and Myf5 are two bHLH transcription factors binding to E-boxes that are important for myogenic differentiation. ChIP-seq analysis for both factors during proliferation and differentiation of primary myoblasts has been reported and reveals that MyoD binds to two sites in the Atp2a1 promoter during myoblast differentiation, whereas Myf5 does not bind under both conditions [39] . We examined binding of MyoD to E-boxes present in the Atp2a1 promoter by ChIP and could confirm strong binding to site X1 and weaker but sigificant binding also to site X5. Also, sites X3 and X4 gave an increased signal, but the values did not reach statistical significance ( Fig. 6b ). In contrast to Ebf3, ChIP-grade antibodies specific for MyoD are available, allowing us to examine its binding in primary diaphragm cells in the presence and absence of Ebf3. 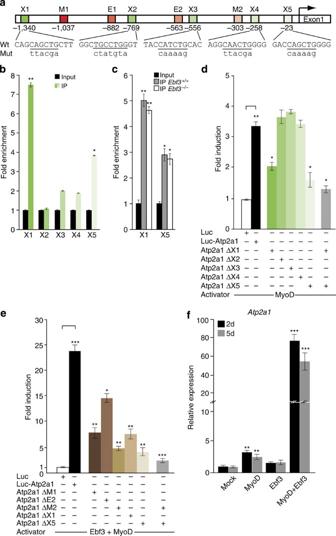Figure 6: Ebf3 synergises with MyoD in the induction of theAtp2a1gene. (a) Schematic overview of the promoter structure of theAtp2a1gene. Ebf consensus sites are indicated in red, E-boxes X1 to X5 in green, and their position relative to the transcriptional start site is shown. The sequence of each potential binding site is indicated, and mutations used in the experiments in this figure are shown in small letters. (b) Chromatin immunoprecipitation (ChIP) of flag-tagged MyoD protein from C2C12 cells; qPCR analysis of ChIP using primers specific for all five individual binding sites. Fold enrichment indicates the ratio of DNA amplification comparing ChIP with beads-only control;n=3; error bars=s.d.; *P<0.05, **P<0.01. (c) ChIP assay of MyoD protein from diaphragm of E18.5Ebf3+/+andEbf3−/−embryos as indicated; qPCR analysis of ChIP using primers specific for the two binding sites determined inb. Fold enrichment indicates the ratio of DNA amplification comparing ChIP with beads-only control;n=3; error bars=s.d.; *P<0.05, **P<0.01. (d) HEK293 cells were transfected with an expression plasmid for MyoD and a reporter construct containing all indicated consensus sites as wild-type or mutated sequence as shown ina, followed by the luciferase gene. Transfections of the pBL-Luc plasmid not containing promoter elements together with pCMV-Ebf3were set to 1 for each reporter plasmid;n=3; error bars=s.d.;P-values were calculated in comparison with activation of pBL-Luc-Atp2a1if not otherwise indicated. *P<0.05, **P<0.01. (e) HEK293 cells were transfected as ind, but expression plasmids for Ebf3 and MyoD were used in parallel, and reporter plasmids with mutations in binding sites were used as indicated. Transfections of the pBL-Luc plasmid not containing promoter elements together with pCMV-Ebf3were set to 1 for each reporter plasmid;n=3; error bars=s.d.;P-values were calculated in comparison with pBL-Luc-Atp2a1if not otherwise indicated. *P<0.05, **P<0.01, ***P<0.001. (f) Quantitative PCR analysis ofAtp2a1expression in C2C12 cells 2 and 5 days after transfection ofEbf3and/orMyoDencoding expression plasmids. Mock (transfection of parental plasmid) is set to 1 for 2 and 5 days.n=3; error bars=s.d.;P-values are relative to mock; **P<0.01, ***P<0.001. Figure 6c confirms binding of MyoD to sites X1 and X5 under wild-type conditions and also shows that MyoD can bind to these sites in the absence of Ebf3. To analyse the functional importance of these E-boxes, we tested them individually with wild-type or mutated sequences together with MyoD. Figure 6d shows that MyoD can transactivate 3.4-fold from the Atp2a1 promoter, which is comparable to the induction with Ebf3 alone. Mutation of the individual E-boxes as indicated in Fig. 6a leads to a reduction in transactivation potential in case of sites X1 and X5 to 2- and 1.8-fold, respectively, whereas sites X2 to X4 have no influence. Combining mutations in sites X1 and X5 leads to a reduction of transactivation to 1.4-fold ( Fig. 6d ). To test potential synergistic effects between Ebf3 and MyoD, we combined these two factors with reporter constructs used before. Together, these two transcription factors lead to a 24.4-fold induction of the Atp2a1 promoter, displaying strong synergy in their transactivation capacity. Mutation of Ebf-binding sites M1 or M2 in this context results in a reduction of transactivation to 7.6-fold and 4.8-fold, respectively, and in a reduction to 14.5-fold in case of site E2 ( Fig. 6e ). E-boxes X1 and X5 are important for co-transactivation, as their mutation reduces induction to 6.8-fold and 4.6-fold. Finally, the combination of the two strongest mutations for each class of transcription factors, M2 and X5, reduced the combined transactivation potential of Ebf3 and MyoD to 2.4-fold ( Fig. 6e ). As Ebf3 alone is not sufficient to induce the expression of endogenous Atp2a1 in C2C12 cells within 2 to 5 days, but can do so in combination with horse serum ( Fig. 5f ), we tested whether Ebf3 and MyoD together have this ability. MyoD alone can induce the expression of Atp2a1 3.2-fold and 2.8-fold after 2 and 5 days, whereas expression of Ebf3 alone does not significantly induce Atp2a1 . Together, however, Ebf3 and MyoD have the potential to strongly induce the expression of Atp2a1 by 74.6-fold and 53.4-fold after 2 and 5 days post-transfection ( Fig. 6f ). The synergistic activity between Ebf3 and MyoD prompted us to investigate a potential direct interaction between these transcription factors. To this end, we transfected C2C12 cells with tagged versions of both factors, and tried co-immunoprecipitation under various conditions, but failed to detect a direct interaction. Figure 6: Ebf3 synergises with MyoD in the induction of the Atp2a1 gene. ( a ) Schematic overview of the promoter structure of the Atp2a1 gene. Ebf consensus sites are indicated in red, E-boxes X1 to X5 in green, and their position relative to the transcriptional start site is shown. The sequence of each potential binding site is indicated, and mutations used in the experiments in this figure are shown in small letters. ( b ) Chromatin immunoprecipitation (ChIP) of flag-tagged MyoD protein from C2C12 cells; qPCR analysis of ChIP using primers specific for all five individual binding sites. Fold enrichment indicates the ratio of DNA amplification comparing ChIP with beads-only control; n =3; error bars=s.d. ; * P <0.05, ** P <0.01. ( c ) ChIP assay of MyoD protein from diaphragm of E18.5 Ebf3 +/+ and Ebf3 −/− embryos as indicated; qPCR analysis of ChIP using primers specific for the two binding sites determined in b . Fold enrichment indicates the ratio of DNA amplification comparing ChIP with beads-only control; n =3; error bars=s.d. ; * P <0.05, ** P <0.01. ( d ) HEK293 cells were transfected with an expression plasmid for MyoD and a reporter construct containing all indicated consensus sites as wild-type or mutated sequence as shown in a , followed by the luciferase gene. Transfections of the pBL-Luc plasmid not containing promoter elements together with pCMV- Ebf3 were set to 1 for each reporter plasmid; n =3; error bars=s.d. ; P -values were calculated in comparison with activation of pBL-Luc- Atp2a1 if not otherwise indicated. * P <0.05, ** P <0.01. ( e ) HEK293 cells were transfected as in d , but expression plasmids for Ebf3 and MyoD were used in parallel, and reporter plasmids with mutations in binding sites were used as indicated. Transfections of the pBL-Luc plasmid not containing promoter elements together with pCMV- Ebf3 were set to 1 for each reporter plasmid; n =3; error bars=s.d. ; P -values were calculated in comparison with pBL-Luc- Atp2a1 if not otherwise indicated. * P <0.05, ** P <0.01, *** P <0.001. ( f ) Quantitative PCR analysis of Atp2a1 expression in C2C12 cells 2 and 5 days after transfection of Ebf3 and/or MyoD encoding expression plasmids. Mock (transfection of parental plasmid) is set to 1 for 2 and 5 days. n =3; error bars=s.d. ; P -values are relative to mock; ** P <0.01, *** P <0.001. Full size image Redundancy between Ebf factors in the induction of Atp2a1 The finding that deficiency for Ebf3 leads to a downregulation of Serca1 in the diaphragm, but not in skeletal muscle, ( Fig. 3h ) is surprising and indicates that either the regulation of Atp2a1 expression is different between these muscle types or that compensation between Ebf proteins is going on. As mentioned in the introduction, Ebf3 is part of a highly homologous family of proteins consisting of four members, of which functional redundancy has already been demonstrated [16] . To analyse whether the mechanism described here might be more general and not restricted to the diaphragm, we isolated RNA from diaphragm and skeletal muscle of wild-type mice and determined the expression of all four Ebf genes by qPCR. Ebf3 shows the strongest expression in the diaphragm, followed by an approximately threefold lower expression of Ebf1 , whereas Ebf2 and Ebf4 are only weakly expressed ( Fig. 7a ). In contrast, Ebf1 is the most strongly expressed family member in the skeletal muscle, Ebf3 is 3.4-fold lower, and Ebf2 and Ebf4 again are only weakly expressed ( Fig. 7b ). To determine whether there is functional redundancy between the individual Ebf factors in the induction of the Atp2a1 gene, we first tested their ability to transactivate from the Atp2a1 promoter. In reporter assays Ebf1, Ebf2 and Ebf4 have a transactivation potential that is comparable to the activity of Ebf3 ( Figs 5d and 7c ), indicating potential redundancy between these factors. To test this ability with the endogenous gene, we ectopically expressed Ebf factors either alone or in combination with MyoD in C2C12 cells and determined the expression of endogenous Atp2a1 after 2 days. Ebf1, Ebf2 and Ebf4 alone can induce the expression of Atp2a1 approximately two- to threefold, again largely recapitulating the ability of Ebf3 alone. In combination with MyoD, however, all Ebf factors show a strong synergistic effect, resulting in a 60- to 80-fold induction of Atp2a1 ( Fig. 7d ). To test these results also genetically, we examined the expression of Atp2a1 in skeletal muscle from Ebf1 wild-type and mutant mice. Loss of one allele of Ebf1 leads to a downregulation of Atp2a1 by 21%, whereas its complete deletion reduces Atp2a1 by 51% ( Fig. 7e ), confirming a more general role for Ebf proteins in its regulation and also indicating dose-dependency of Ebf factors in the induction of the Atp2a1 gene. 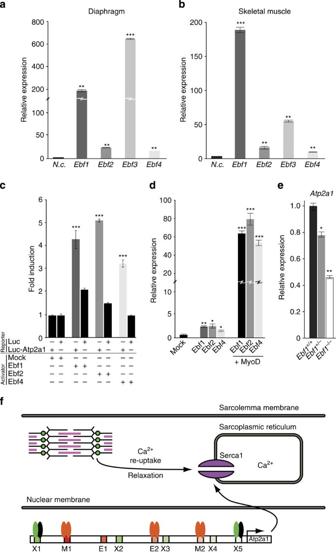Figure 7: Overlapping expression and redundancy between Ebf genes. (a) Expression of Ebf factors as indicated in the diaphragm from E18.5 embryos determined by quantitative PCR. Ba/F3 cells were used as negative control (n.c.).n=3, error bars=s.d., **P<0.01, ***P<0.001. (b) Same asa, but skeletal muscle from adult mice was used for analysis.n=3, error bars=s.d., **P<0.01, ***P<0.001. (c) Analysis of the transactivation potential of Ebf factors from theAtp2a1promoter. HEK293T cells were transfected with reporter plasmids comprising all four Ebf consensus sites in wild-type form as inFig. 7d. Ebf1, Ebf2 and Ebf4 in pCMV were co-transfected as activators as indicated. Transfections of the empty pCMV plasmid were set to 1, and all other values are given accordingly.n=3, error bars=s.d., ***P<0.001,P-values are in comparison with mock control of the respective reporter. (d) Analysis of the expression ofAtp2a1in C2C12 cells by qPCR in response to ectopic expression of Ebf1, Ebf2, Ebf4 and MyoD as indicated 2 days after transfection.n=3, error bars=s.d., *P<0.05, **P<0.01, ***P<0.001. (e) Expression ofAtp2a1determined by qPCR from skeletal muscle ofEbf1+/+,Ebf1+/−andEbf1−/−mice (E18.5);n=3, error bars=s.d., *P<0.05, **P<0.01. (f) Model for the role of Ebf factors in muscle physiology. Ebf (orange ovals) and MyoD (green ovals) directly bind to consensus sequences present in the promoter of theAtp2a1gene and synergistically transactivate the expression ofAtp2a1. Serca1 mediates Ca2+re-uptake and muscle relaxation, which are defective in absence ofEbf3. Figure 7: Overlapping expression and redundancy between Ebf genes. ( a ) Expression of Ebf factors as indicated in the diaphragm from E18.5 embryos determined by quantitative PCR. Ba/F3 cells were used as negative control (n.c.). n =3, error bars=s.d., ** P <0.01, *** P <0.001. ( b ) Same as a , but skeletal muscle from adult mice was used for analysis. n =3, error bars=s.d., ** P <0.01, *** P <0.001. ( c ) Analysis of the transactivation potential of Ebf factors from the Atp2a1 promoter. HEK293T cells were transfected with reporter plasmids comprising all four Ebf consensus sites in wild-type form as in Fig. 7d . Ebf1, Ebf2 and Ebf4 in pCMV were co-transfected as activators as indicated. Transfections of the empty pCMV plasmid were set to 1, and all other values are given accordingly. n =3, error bars=s.d., *** P <0.001, P -values are in comparison with mock control of the respective reporter. ( d ) Analysis of the expression of Atp2a1 in C2C12 cells by qPCR in response to ectopic expression of Ebf1, Ebf2, Ebf4 and MyoD as indicated 2 days after transfection. n =3, error bars=s.d., * P <0.05, ** P <0.01, *** P <0.001. ( e ) Expression of Atp2a1 determined by qPCR from skeletal muscle of Ebf1 +/+ , Ebf1 +/− and Ebf1 −/− mice (E18.5); n =3, error bars=s.d., * P <0.05, ** P <0.01. ( f ) Model for the role of Ebf factors in muscle physiology. Ebf (orange ovals) and MyoD (green ovals) directly bind to consensus sequences present in the promoter of the Atp2a1 gene and synergistically transactivate the expression of Atp2a1 . Serca1 mediates Ca 2+ re-uptake and muscle relaxation, which are defective in absence of Ebf3 . Full size image Taken together, the data show that Ebf3 is necessary for the relaxation of the diaphragm by binding to three consensus sites in the promoter/enhancer of the Atp2a1 gene, where it synergises with MyoD to induce the expression of Serca1, which is necessary for Ca 2+ -uptake into the sarcoplasmic reticulum ( Fig. 7f ). This mechanism, however, is not restricted to Ebf3 and the diaphragm but general in muscle cells as all Ebf factors can synergise with MyoD and transactivate from the Atp2a1 promoter. An overlapping, but also distinct expression pattern, between mostly Ebf1 and Ebf3 in the diaphragm versus the skeletal muscle is responsible for biological effects. The transcription factor Ebf3 was originally identified because of its expression in the olfactory epithelium and neuronal cells [18] , [19] , and Ebf3 -deficient mice have defects in olfactory receptor neuron projection [16] . However, Ebf3 is also expressed outside of the neural system and Ebf3 −/− mice die immediately after birth, but only very little is known about its role in other tissues. Here, we identify respiratory failure caused by the inability of the lung to unfold at birth as the reason for the postnatal death. Multiple organs might account for such a phenotype, including the lung, the rib cage and the muscles involved in respiration, that is, mainly the diaphragm and the heart. Ebf3 is not expressed in the lung and the heart, and development of the lung, heart and bone proceeds normally in the absence of Ebf3 . However, Ebf3 is expressed strongly in the diaphragm, suggesting an involvement of muscle cells in the Ebf3 -dependent respiratory failure. Consistent with this notion, the function of Ebf3 -deficient muscle cells of the diaphragm is impaired, resulting in less force produced in response to single or persistent stimulation and prolonged duration of muscle contraction after stimulation. This phenotype of impaired muscle relaxation is highly reminiscent of the deletion of Atp2a1 , which encodes for a Ca 2+ -ATPase that catalyses the ATP-dependent transport of Ca 2+ from the cytosol to the lumen of the sarcoplasmic reticulum [40] . Interestingly, Serca1 is strongly downregulated in the diaphragm but not in skeletal muscle of Ebf3 -deficient mice. Ebf1 , a highly homologous member of this family of transcription factors, is most strongly expressed in skeletal muscle. Ebf1 can act via the same binding sites in the Atp2a1 promoter, synergises with MyoD, and loss of Ebf1 leads to a downregulation of Atp2a1 expression in skeletal muscle, indicating redundancy between individual Ebf factors. It is an interesting question why the diaphragm differs in its expression of Ebf factors from other skeletal muscles, however, as the promoters of Ebf genes have not been characterized with the exception of Ebf1, this remains subject for further study. An important question is also why there is a downregulation of Atp2a1 in the absence of Ebf3 since Ebf1 is expressed in the diaphragm as well and is also able to induce its expression. Ebf factors have dose-dependent effects in other cellular contexts like B-cell and neuronal development [16] , [35] and, in fact, deletion of only one allele of Ebf1 also leads to a slight reduction of Atp2a1 in skeletal muscle. Therefore, dose dependency seems to be responsible for this effect. The large phenotypic overlap between loss of Ebf3 and Atp2a1 is striking and together with its downregulation already indicates the potential importance of Atp2a1 as a target gene of Ebf3. The genetic rescue of Ebf3 -dependent muscle relaxation and respiratory failure by ectopic expression of Atp2a1 in vivo identifies it as the biologically most relevant downstream target of Ebf3 in the diaphragm. However, Serca1 does not completely rescue deficiency for Ebf3 as mice die within 4 days after birth. This is likely the result of a complex situation in the compound Ebf3/Atp2a1 mutant animals. The skeletal α-actin promoter does not recapitulate the expression pattern of the endogenous Atp2a1 promoter, and in addition the expression of Atp2a2 is strongly downregulated. We failed to identify Ebf-binding sites in the promoter/enhancer of the Atp2a2 gene, and ectopic expression of Ebf3 and MyoD alone or in combination did not alter Atp2a2 expression levels in C2C12 cells. In addition, since Atp2a2 is expressed in slow twitch fibres, its downregulation seems to be indirect. As this situation is not only complex, but due to the expression of the transgene to some degree also artificial, we decided not to follow the synthetic phenotype any further. Therefore, the analysis of the biological role of Ebf3 after birth awaits the generation of conditional knock-out mice. Interestingly, many muscle-specific genes harbour E-boxes in their promoter, which act as binding sites for MRF proteins [4] , [7] . However, E-boxes are not tissue-specific as they occur not only in muscle-specific genes, but also have a much broader distribution, and MRF factors bind to many E-boxes in nonmuscle-specific promoters [8] . Consequently, an important question in muscle development is how specificity is achieved. A combinatorial action between MRF and other transcription factors has been suggested, and a few examples have been identified [10] , [41] . In B-cell development, Ebf1 acts synergistically with the transcription factor E47, a product of the E2A gene, which also binds to E-boxes [35] . Although no direct interaction could be demonstrated so far, they cooperate in the induction of B-cell-specific genes [36] . There are several striking parallels to the data presented here, like the involvement of Ebf factors and E-box binding proteins, direct binding to neighbouring sites in the promoter, no detectable physical interaction but cooperation in the induction of the downstream gene. Furthermore, MyoD can replace products of the E2A gene in the synergistic induction of the B-cell-specific lambda5 gene, demonstrating redundancy between bHLH transcription factors in the cooperation with Ebf proteins [42] . Therefore, synergistic effects between E-box-binding factors and Ebf proteins seem to be a broader phenomenon and not restricted to B cells. Consequently, although Ebf3 just as other Ebf factors is clearly not muscle specific, it could be part of a transcriptional module that together mediates muscle-specific gene expression. In parallel to the high conservation of Ebf genes at the sequence level during evolution [13] , [14] , [43] , there seems to be also a considerable level of conservation of their biological role. Collier , the only Ebf gene in Drosophila, is expressed by cells that support immature haemocytes and is necessary to maintain this pool of progenitor cells [44] . This is highly reminiscent of Ebf2 and its role in the support of immature haematopoietic stem and progenitor cells [45] . Besides the support of haemocytes, collier is also required for the formation of the dorsal/acute 3 (DA3) embryonic muscle, which does not develop in its absence [46] , [47] . Together with nautilus , the only homologue of MRF bHLH factors in Drosophila, collier controls shape and morphology of the DA3 muscle [48] . Here we report that Ebf3 is required for the relaxation of the diaphragm and that it synergises with MyoD in inducing a critical cell-type specific gene. To our knowledge this is the first implication of Ebf genes in muscle cell function in mammals, but the phenotype described here differs considerably from the loss of collier in Drosophila. Hence, either the requirement for Ebf factors has changed during evolution or the expression of other Ebf family members and redundancy might mask a broader role for this gene family in muscle development. Indeed, it was recently shown that Ebf proteins participate in transcriptional regulation of muscle development in Xenopus [49] , favouring the second possibility. In parallel to a strong evolutionary conservation at the sequence level, there might be also a conservation at the level of interaction partners like bHLH transcription factors. Although collier and Ebf3 are required for development and function of a specific muscle, such a conservation seems true at the broad biological level, but not in detailed aspects. The diaphragm is a derivative of myoblasts from myotomes C3, C4 and C5, which migrate into the septum transversum, a condensation of mesenchymal cells pre-figuring large parts of the diaphragm, where they expand and differentiate. This process is not homologous to the generation of the DA3 muscle, but it is tempting to speculate that a conservation in the specification of muscle identity might exist at the molecular level despite different organ development at the cellular level. Therefore, rather than postulating a relationship between the DA3 muscle in Drosophila and the diaphragm in the mouse, it seems more likely that Ebf factors probably in combination with the E-box-binding MRF factors form a module in muscle cell differentiation that has been adopted during evolution. Brody’s disease is a rare myopathy, characterized by exercise-induced impairment of skeletal muscle relaxation, stiffness and cramps, resulting from impaired Ca 2+ -uptake and Ca 2+ -ATPase activity [50] . Mutations of Atp2a1 were found in 50% of Brody’s patients and are genetically associated with Brody disease [51] . The reason for the remaining cases of Brody myopathy is unclear, as the genomic sequence of Atp2a1 is unchanged. Among these, cases have been reported in which the expression of Serca1 is strongly reduced [52] . As Serca1 is strongly downregulated and barely detectable in the diaphragm of Ebf3 -deficient mice, we suggest that Ebf3 might be involved in at least a subgroup of the remaining cases of Brody disease. This might be either via mutation of Ebf3 itself, but this is the more unlikely possibility as the broad expression of Ebf3 will probably result in more defects after birth. Alternatively, binding sites for Ebf proteins might be mutated, preventing Ebf3 from transactivating from the human Atp2a1 promoter. Generation of mice Two DNA fragments corresponding to the Ebf3 genomic region were isolated from a mouse 129/Ola genomic cosmid library. The first fragment (5′-region) expanded 4.85 kb from a PmlI site upstream of the Ebf3 coding region to the translation start codon. The second region was a PstI fragment of 4.6 kb from intron 4 to intron 6. The targeting construct was obtained by cloning these fragments in the pBluescript KS vector, followed by insertion of an NLS-lacZ gene and a PGK::Neo cassette flanked by loxP sites between both fragments. NLS-LacZ was cloned in frame with the Ebf3 translation start codon. Mouse ES cells were electroporated with this construct, and colonies were isolated in the presence of 400 μg ml −1 G418. For DNA extraction, cells were digested with 100 μg ml −1 Proteinase K in the presence of 50 mM Tris-HCl pH 7.5, 100 mM NaCl and 10% SDS. DNA was ethanol precipitated and analysed by Southern Blot [53] . Two clones (#1 and #2) out of the 800 clones analysed had correctly incorporated the targeting construct, as established by Southern blot. Both clones were injected into C57BL/6 blastocysts that were implanted into pseudopregnant females. Chimeric mice were bred to obtain germline transmission. Two male chimera (80%) corresponding to clone #1 were selected to get heterozygous mice. The PGK::Neo cassette was removed by crossing with PGK-Cre transgenic mice [54] . Mutant mice were backcrossed with C57Bl/6 wild-type mice for more than 10 generations. All experiments involving animals were designed in agreement with the stipulations of the animal care committee of the Helmholtz Zentrum München and the ‘Regierung von Oberbayern’. Genotyping For genotyping of mice tails were digested for at least 1 h in lysis buffer (FirePol buffer B (Solis BioDyne), 1.25 mM MgCl 2 , 50 μg ml −1 proteinase K) at 55 °C and inactivated for 15 min at 95 °C. PCR was carried out with genomic DNA and 20 pmol of each primer ( Ebf3 fwd 5′-GGGCACACCACAGTCTGTC-3′, Ebf3 wt rev 5′-GGAGGATATACAGGGTCACAC-3′, Ebf-lacZ rev 5′-GCGCCGGTCACCATTACC-3′) using FirePol (Solis BioDyne) under these conditions: 35 cycles of 94 °C for 30 s, 61 °C for 1 min, 72 °C for 30 s. Atp2a1 -transgenic mice were obtained from Jeffery Molkentin (University of Cincinnati, USA) and genotyped as described [30] . Isolation of primary cells Bone marrow cells were isolated as described [55] . For isolating bone marrow cells, bones (two tibia and two femurs per mouse) from embryos at day E18.5, bones were pre-digested in DMEM supplemented with 0.1% collagenase (Sigma) and 0.2% dispase (Roche) twice for 20 min. After washing with PBS, bones were cut and digested three times as above, and supernatant was collected. For cell isolation from whole organs, adult or embryonic mice were killed, organs removed and detached by a 100-μm cell strainer. Diaphragm cells were digested in DMEM supplemented with 0.2% collagenase for 30 min, fractionated and resuspended. Electrophysiology and force measurements Experiments were conducted on diaphragm muscle strips from newborn mice. The pups were killed by cervical dislocation and after the laparotomy, the rib cage containing the whole diaphragm was excised and kept in cold MEM-Glutamax (Gibco) supplemented with fetal bovine serum for dissection. A strip from the right ventral costal hemi-diaphragm was excised keeping both insertions from ribs and central tendon intact. The muscle strips were horizontally mounted in Ringer-Krebs-Henseleit solution (140 mM NaCl, 5 mM KCl, 1.2 mM KH 2 PO 4 , 1.2 mM MgCl 2 , 2 mM CaCl 2 , 20 mM Hepes, 6 mM glucose; pH 7.4; osmolarity between 290–315 mOsM). At constant perfusion, the solution was kept at 25 °C and bubbled with gas mixture of 95% O 2 and 5% CO 2 . The costal end was held in a stationary end and the central tendon attached to the force transducer (SI-H Force Transducer, 0–50 mN, SI-KG4, WPI). The optimal length (Lo) was defined as the muscle length at which twitch tension development was maximal, corresponding to the apex of the length-active tension curve. Stimulation was applied using a Grass stimulator SD9 (Grass Instruments, Quincy, MA) via closely flanking platinum wire electrodes. Supramaximal stimulation during single twitch was reached at 50 V, with 1 ms squared pulse duration. Duration of tetanus stimulation was set for 500 ms. The diaphragm force-frequency relationship was assessed at supramaximal stimulation by sequential excitation of muscles at 50 V with pulse duration of 1 ms at 1, 5, 10, 15, 30, 60, 90, 120, 150 and 180 Hz, during 500 ms, every 3 min. The cross-sectional area (CSA) of the muscle strip was calculated by dividing the mass of the muscle (without rib bone and central tendon; mg) by the product of the optimal length (Lo, mm) and muscle density (1.056 g cm −3 ). The tension was calculated as force (mN) per CSA (cm 2 ). The traces were acquired at 4 KB s −1 and analysed using PowerLab and LabChart 7.0 (AD Instruments, Australia). Cell Culture 70Z/3, 18-81 TK+ and Ba/F3 cells were cultured in RPMI 1640, supplemented with 10% fetal calf serum (FCS; PAA), 1% penicillin and streptomycin, 1% L -glutamine. For 70/Z3 and 18-81 TK+, 1% sodium pyruvate and 0.003% β-mercaptoethanol was used additionally. For the maintenance of Ba/F3 cells, the culture medium was supplemented in addition with 10% conditioned medium from WEHI3 cells as a source of IL-3. WEHI-3B and Whitlock-Witte cultures were propagated in RPMI 1640 supplemented with 10% FCS and 0.0003% β-mercaptoethanol. Stromal cell lines (2018, AFT024, C2C12, GP+E86, HEK293T) were grown in Dulbecco’s modified Eagle medium with Glutamax (DMEM), and osteoblastic cells (C3H10T½, MC3T3) were cultured in minimum essential medium (MEMalpha) with in addition supplemented 10% FCS, penicillin and streptomycin and L -Glutamine. All reagents described were purchased from Gibco unless stated otherwise. In vitro differentiation assay was performed as described [56] . In brief, C2C12 cells were transfected with Ebf3 -expressing plasmid, and in vitro differentiation was initiated by adding 2% horse serum in medium instead of fetal calf serum for 2 or 5 days. CFU-F assay Mouse bone marrow cells were harvested from E18.5 Ebf3 +/+ and Ebf3 −/− mice as described above. Cell numbers were determined by using Casy cell counter (Schärfe Systems). Cells were diluted in mouse Complete MesenCult Medium (StemCell Technologies), and 10,000 cells were seeded per well in six-well plates. The cells were cultured at 37 °C in 5% CO 2 for 10 days without medium change. The medium was aspirated, and each well was washed twice with PBS thereafter. Cells were fixed with methanol for 10 min at room temperature. The methanol was removed, and each well was stained with Giemsa Staining Solution for 10 min at room temperature. The staining solution was aspirated and each well was washed with water for several times to remove unbound stain. The water was removed and the wells were allowed to air dry. Stained colonies were counted microscopically. Electron microscopy Mice were killed at indicated embryonic days. After fixating whole mice in fixation buffer (2.5% PFA, 2% glutaraldehyde, Sörens-buffer (pH 7.4)) for 1 h, further fixation of single organs was carried out in 2.5% glutaraldehyde at 4 °C. Samples were washed three times with cacodylate buffer (pH 7.4, Science Services) and fixated in chromosmium acid (1.25% potassium dichromate (K 2 Cr 2 O 7 ; pH 7.2), 1% osmium tetroxide (OsO 4 ), 0.85% NaCl). After stepwise dehydration, samples were treated with propylenoxide (Merck). Afterwards, samples were incubated in 1:11-mixture (Epon (246 mg ml −1 dodecenylsuccinic anhydride (Merck), 326 mg ml −1 methyl-5-norbornene-1,3-dicarboxylic anhydride (Roth), 522 mg ml −1 glyicidyl ether 100 (Epon 812, EMS), 15 μl ml −1 2,4,6-tris-dimethylaminomethyl-phenol (Roth) and propylene oxide (Merck)). Sections were generated using Leica Ultramicrotome and stained with haematoxylin/eosin or analysed by using a transmission-electron microscope EM 10 CR (Zeiss). Haematoxylin/eosin staining Sections were hydrated and afterwards incubated for at least 4 h in haematoxylin buffer (0.2 g l −1 sodium iodate, 91.8 g l −1 potassium alum sulphate, 50 g l −1 chloralhydrate, 1 g l −1 citric acid, 1 g l −1 hematoxylin; Merck). Following a washing step with water, sections were stained for 20 s with Eosin (0.17% acid, 0.58% sodium acetate, 5 g l −1 eosin Y; Merck) and washed again. For mounting, sections were again stepwise dehydrated, incubated with xylene and embedded with Eukitt (Kindler). β-Galactosidase staining Cryosections or whole embryos were perfused in phosphate buffer (23 mM sodium phosphate monobasic, 77 mM sodium phosphate dibasic, pH 7.3). After fixation (0.2% glutaraldehyde, 0.5 mM EGTA (pH 7.3), 2 mM magnesium chloride, 94 mM sodium phosphate (pH 7.3)), samples were washed three times in wash buffer (625 M magnesium chloride, 0.02% Nonidet-P40, 97.6 mM sodium phosphate, pH 7.3). Staining was carried out in staining solution (96% wash buffer as mentioned above, 4% di-methyl formamide, 10 mg ml −1 X-gal (Roche), 2.12 mg potassium ferrocyanide, 1.64 mg potassium ferricyanide) for at least 16 h. Samples were washed as above, fixed with 4% PFA, washed twice in PBS and stepwise dehydrated. After incubation in xylene, sections could be mounted (DPX Mountant, Fluka). All reagents were obtained from Sigma, if not otherwise provided. Whole mounts were stained as described above, but were photographed after fixing and washing steps. Bone histology Analysis of bone and cartilage by alcian blue/alizarin red staining was done as described [27] . In brief, skin of the embryo was removed and whole embryo was fixed in 95% ethanol for several days. All internal organs were removed and skeletal tissue was stained for at least 18 h using alcian blue (90% ethanol, 20% glacial acetic acid, 0.19 mg ml −1 alcian blue). After washing twice with 95% ethanol, embryos were macerated in 2% potassium hydroxide. Next, embryos were stained with Alizarin Red S in 2% KOH solution. After stepwise dehydration of the embryo in KOH-glycerine solution, skeleton and cartilage were analysed. To examine calcified bone matrix, femurs and tibia from embryos were cryosectioned and stained by von Kossa solution as described [27] . Flow cytometry For flow cytometry, cells were obtained from the diaphragm or the bone marrow as described above. Isolated cells were incubated with fluorochrome-conjugated antibodies according to standard procedures, measured or sorted using either a FACSCalibur or a FACSAriaIII (BD Biosciences), and data were analysed using CELLQuestPro, FACSDiva Software (Becton Dickinson GmbH) and FlowJo 9.3 (Treestar) software. For depletion of dead cells propidium iodide was used. Conjugated antibodies directed against the following markers were obtained from BD Biosciences: Mac1 (M1/70), Gr1 (RB6-8C5), B220 (RA3-6B2) and CD43 (RM4-5). Antibody CD45.2 (104) was obtained from eBioscience. All antibodies were used at a dilution of 1:250. For Ebf3-β-galactosidase detection, cells were isolated as described above, incubated in 1% FCS and 1 mM fluorescein digalactoside (FDG; Invitrogen) for 75 s at 37 °C and resuspended in ice-cold DPBS thereafter. Gene expression analysis measurement by qPCR In brief, mRNA was isolated from cells, whole organs or embryos using peqGOLD TriFast (Peqlab) according to manufacturer’s instructions; organs and embryos were dispersed before using an Ultra Turrax T25 (IKA Labortechnik). cDNA was synthesized with a SuperScript II reverse transcriptase kit (Invitrogen). PCR reactions were performed in duplicate with SYBR Green I Master in a LightCycler 480II (Roche) with standard conditions: 95 °C for 10 min followed by 45 cycles of 95 °C for 10 s, 65 °C for 10 s and 72 °C for 10 s. Alternatively, 40 cycles with an annealing temperature of 63 °C were used. Primer sequences for Atp2a1a+b, Atp2a 2a, Atp2a 2b, Atp2a 1 + 2, Atp2a 2, Atp2a 3, Sarcolipin and Phospholamban are described [29] ; sequences for MyHC-I β , MyHC-IIA, MyHC-IIB, MyHC-IIX/D are according to [57] , and all other sequences are listed in the Supplementary Methods . Target gene expression was normalized to Hypoxanthine phosphoribosyltransferase ( HPRT ) expression. Cloning and site-directed mutagenesis Ebf3 was inserted into the mammalian expression vector pCMV cyto using standard methods. CTAP-MyoD was obtained from Michael Rudnicki (University of Ottawa, Canada) as described [39] . PCR using specific primer for genes or genomic DNA were designed with additional restriction sites as indicated below with italic letters. Subcloning was done by digesting PCR products and relevant vectors with corresponding enzymes for at least 3 h, purified by gel extraction kit (Qiagen), and ligated for at least 16 h at 16 °C. The QuikChange site-directed mutagenesis kit (Stratagene) was used according to the manufacturer’s instructions to introduce mutations into Ebf-binding sequences. Primer sequences to generate point mutations are indicated with small letters given below; binding site core palindromes are underlined. Sequencing was done for each construct to exclude errors. Protein extraction and western blotting Cells or organs were washed twice in ice-cold PBS and solubilised in the lysis buffer (50 mM Tris (pH 8), 150 mM NaCl, 1% NP-40, 1 μg ml −1 leupeptin, 1 μg ml −1 aprotinin, 100 μg ml −1 PMSF] using Ultra Turrax T25. The samples were lysed for 40 min on ice. The supernatant (soluble whole-cell lysate) was fractionated on a 10-12% SDS-polyacrylamide gel and then transferred onto nitrocellulose membranes (Protran, Whatman). Membranes were first blocked in 5% milk-PBS-Tween and then incubated for 14 h at 4 °C with 5% milk-PBS-Tween containing the first antibody in a dilution recommended by the manufacturer. Membranes were washed three times with PBS-Tween, incubated with 5% milk-PBS-Tween, containing alkaline phosphatase-conjugated secondary polyclonal antibody, and then washed as mentioned above. Signals were detected using detection mixture (0.1M Tris-HCl (pH 8.6), 0.25 mg ml −1 luminol, 0.11 mg ml −1 para-hydroxy-conmarin acid, 0.009% H 2 O 2 ) and Hyperfilm ECL (Amersham). The anti-β-Actin (AC-74), α-Flag (M2; F3165), α-Serca1 (adult; IIH11) and secondary α-mouse-IgG.HRP antibodies were obtained from Sigma. The anti-β-Tubulin (5H1) was obtained from BD Pharmingen and α-Serca1 (embryonic; VE121G9) antibody from Thermo Scientific. The secondary α-rat-IgG+IgM.HRP antibody was purchased from Jackson Immuno Research. Bands in western blot experiments were quantified using the open source software ImageJ ( http://rsb.info.nih.gov/ij/ ; W. S. Rasband, NIH, National Institutes of Health, Bethesda, MD). Statistics P -values were determined with the Student’s two-tailed t-test for independent samples, assuming equal variances on all experimental data sets. EMSA Double-stranded oligonucleotides were annealed in annealing buffer (10 mM Tris/HCl (pH 7.4), 10 mM MgCl 2 , 50 mM NaCl) and labelled by filling up with Klenow enzyme, [α-P 32 ]-dCTP, and unlabelled dATP, dGTP and dTTP and purified using Sephadex G50 columns (Amersham Bioscience). The probes used, are listed below. Probes with mutations (small letters) in Ebf-binding sites (underlined) were synthesized as shown in Fig. 6a . EMSA was performed as following: 5 μg protein extracts from HEK293T cells (as described in protein extraction) was mixed in either binding buffer 1 (10 mM HEPES (pH 7.9), 70 mM KCl, 4% glycerol, 1 mM EDTA, 1 mM DTT, 1 × protease-inhibitor (complete mini EDTA-free, Roche), 2 μl poly(dIdC) (1 mg ml −1 , Sigma), 2 μl BSA (1 mg ml −1 ), 2.5 mM MgCl 2 ) or for M2-binding site in binding buffer 2 A(20 mM HEPES (pH 7.9), 75 mM NaCl, 1% glycerol, 1 μg ml −1 salmon sperm DNA, 2 mM DTT, 1 × protease-inhibitor (complete mini EDTA-free, Roche), 1 μl poly(dIdC) (1 mg ml −1 , Sigma) 2 μl BSA (1 mg ml −1 ), 2 mM MgCl 2 ) with either wild-type or mutated probe DNA (250 ng μl −1 ), anti-Flag M2 (F3165; Sigma) antibody or 10-fold concentrated unlabelled probe for competition as indicated. Binding complexes were fractionated on a 4% polyacrylamide gel. After drying of the gel, signals were detected using Biomax MS films (Kodak). Chromatin Immunoprecipitation For ChIP assay, either C2C12 cells were transiently transfected for 2 days or single-cell suspensions of 10 diaphragms of Ebf3 +/+ and Ebf3 −/− mice each were pooled, resuspended in IP-Buffer (10 mM Hepes (pH 7.9), 10 mM KCl, 1.5 mM MgCl 2 , 0.34 M sucrose, 10% protein inhibitors (complete mini EDTA-free, Roche) in glycerol, 0.1% Triton X-100) and partially digested in 1,000 U Mnase (NEB) for 2 min at 37 °C. Mnase was inactivated by adding 10 mM EGTA. Afterwards, 150 mM KCl and 0.2% TritonX-100 were added and immunoprecipitation was performed with α-Flag-coupled magnetic beads (M2; Sigma) or an α-MyoD specific antibody (5.8A, Santa Cruz Biotechnology) for at least 16 h at 4 °C under rotation. Then samples were washed twice with washing buffer A (50 mM Hepes (pH 7.9), 140 mM NaCl, 1 mM EDTA, 1% Triton X-100, 0.1% Na-deoxycholate, 0.1% SDS) and twice with washing buffer 2 (washing buffer 1, 500 mM NaCl) for 10 min. Precipitated complexes were eluted in elution buffer (50 mM Tris (pH 8.0), 1 mM EDTA, 1% SDS), reverse crosslinked by incubation at 65 °C for at least 16 h and purified using NucleoSpin PCR purification kit (Macherey-Nagel). DNA was used for RT–PCR as indicated above, and oligonucleotides and PCR programme are listed above. Input samples were amplified simultaneously to internal controls. Transient transfections and reporter assay C2C12 cells were transfected by Lipofectamine 2000 (Invitrogen) as described in manufacturer’s protocol with a 1:3 ratio of DNA (μg) and Lipofectamine (μl). HEK293T cells were transfected using polyethylenimine (PEI, 1mg ml −1 ; Sigma) according to the standard conditions with a 1:1 ratio of DNA (μg) and PEI (μl). For reporter assays, HEK293T cells were transfected with 5 μg of plasmid DNA (composed of reporter/luciferase (pCMVcyto), activator (pBLLuc5) and β-Galactosidase (pCMVlacZ) plasmids; 5:10:1). Cells were harvested in 100 μl reporter lysis buffer (10% glycerol, 1% Triton X-100, 2 mM EDTA, 25 mM Tris (HCl; pH 7.8), 2 mM DTT) 48 h post-transfection. Measurement of luciferase activity was carried out by adding assay buffer (20 mM tricin, 1.07 mM magnesium carbonate pentahydrate, 2.67 mM MgSO 4 , 33.3 mM DTT, 0.1 mM EDTA, 530 μM ATP, 270 μM acetyl-coenzyme A, 470 μM D(−)-luciferin (Roche), pH 5.8) to the sample duplicates at 560 nm in the micro-plate luminometer OrionII. β-Galactosidase activity was measured at 475 nm after adding first assay buffer (1% Tropix GalactonPlus; Applied Biosystems, 1 mM MgCl 2 , 100 mM Na-P pH 8) and 20 min later activation buffer (0.2 M NaOH; 10% Tropix Emerald Enhancer; Applied Biosystems). How to cite this article: Jin, S. et al . Ebf factors and MyoD cooperate to regulate muscle relaxation via Atp2a1 . Nat. Commun. 5:3793 doi: 10.1038/ncomms4793 (2014).